α-Tanycytes of the adult hypothalamic third ventricle include distinct populations of FGF-responsive neural progenitors Emerging evidence suggests that new cells, including neurons, can be generated within the adult hypothalamus, suggesting the existence of a local neural stem/progenitor cell niche. Here, we identify α-tanycytes as key components of a hypothalamic niche in the adult mouse. Long-term lineage tracing in vivo using a GLAST::CreER T2 conditional driver indicates that α-tanycytes are self-renewing cells that constitutively give rise to new tanycytes, astrocytes and sparse numbers of neurons. In vitro studies demonstrate that α-tanycytes, but not β-tanycytes or parenchymal cells, are neurospherogenic. Distinct subpopulations of α-tanycytes exist, amongst which only GFAP-positive dorsal α2-tanycytes possess stem-like neurospherogenic activity. Fgf-10 and Fgf-18 are expressed specifically within ventral tanycyte subpopulations; α-tanycytes require fibroblast growth factor signalling to maintain their proliferation ex vivo and elevated fibroblast growth factor levels lead to enhanced proliferation of α-tanycytes in vivo. Our results suggest that α-tanycytes form the critical component of a hypothalamic stem cell niche, and that local fibroblast growth factor signalling governs their proliferation. Adult neural stem cell niches, harbouring neural stem and progenitor cells and supporting adult neurogenesis, have been well described in the subventricular zone (SVZ) of the lateral ventricles and the subgranular zone (SGZ) of the hippocampal dentate gyrus. In addition, in vivo analyses show constitutive proliferation, neurogenesis and astrocyte generation within a third region of the adult brain, the hypothalamus [1] , [2] , [3] , [4] , [5] . Here, neurogenesis and gliogenesis can be attenuated through the manipulation of secreted trophic factors, de novo neurogenesis, in particular, associated with energy balance [1] , [2] , [4] , [6] , [7] . The precise location, identity and potential of adult hypothalamic stem/progenitor cell(s), however, remain unclear. Within the adult hypothalamus, cells around the third ventricle form neurospheres (a hallmark of neural stem cells (NSCs) [8] , [9] , [10] ). These studies have raised the possibility that the adult hypothalamus contains NSCs in a niche near the third ventricle. However, tanycytes, ependymocytes, subventricular astrocytes and parenchymal glial cells all reside near the third ventricle, and each is a potential adult stem and progenitor cell candidate [2] , [5] , [6] , [7] , [8] , [11] , [12] , [13] . Hypothalamic tanycytes resemble embryonic radial glia, with a cell body at the ventricular zone and a long basally extending process, their morphology well-suited to their postulated role as modulators of neuroendocrine activity and homeostasis (reviewed in [13] , [14] , [15] , [16] ). Within the hypothalamus, tanycyte cell bodies are strictly localised to the central and posterior hypothalamus (level of the median eminence and premammillary nucleus, respectively). Here they constitute the main cell type lining the ventral third of the third ventricle, interdigitating with ciliated ependymal cells that lack a basal process (ependymocytes) more dorsally [17] , [18] , [19] , [20] , [21] . Morphological studies have mapped and defined subpopulations of tanycytes according to their position and process projection. Ventral-most β-tanycytes line the infundibulum and median eminence, while adjacent α-tanycytes line regions of the ventricular zone (VZ) that are adjacent to hypothalamic nuclei and project laterally, contacting capillaries and neurons of the arcuate and ventromedial nuclei en passant [14] , [18] , [19] . Increasing numbers of studies have focused attention on tanycytes as potential adult NSCs. In the adult rat, fate-mapping experiments of the hypothalamic ventricular wall first showed that proliferating ependymal cells, including but not exclusively tanycytes, can give rise to progeny that migrate along tanycyte processes [11] . Additional studies in the adult rat revealed an enhanced proliferation of tanycytes in response to IGF-1 [6] . In the mouse, lineage-tracing studies have demonstrated that a subset of β-tanycytes, the β2-tanycytes, can proliferate and are neurogenic, contributing new neurons to hypothalamic nuclei in the postnatal/juvenile period [22] . Furthermore, a recent complementary study suggests that ventrally located tanycytes, including β-tanycytes, can proliferate in early adulthood, giving rise to new neurons [23] . However, in contrast to the SVZ of the lateral ventricle wall [24] , lineage-tracing studies have not yet identified a self-renewing multipotent neural stem-like cell in the adult. It remains unclear, moreover, if adult tanycytes have stem-like or progenitor-like activity; indeed it is unknown if adult tanycytes are homogeneous in terms of their neural precursor status. These questions, and the question of the extent of activity of adult tanycytes, remain a challenge. Employing a range of in vitro and in vivo approaches, we demonstrate that in the adult mouse, α-tanycytes lining the third ventricle have NSC characteristics. Lineage-tracing experiments using GLAST::CreER T2 mice provide compelling evidence that GLAST + α-tanycyte cells can self-renew, and constitutively give rise to other tanycyte subclasses, parenchymal astrocytes and neurons, the long tanycyte processes potentially providing a migration route for newborn cells. However, the sparse numbers of neurons that we observe suggests that α-tanycytes are not overtly neurogenic in the unchallenged adult mouse. We show, further, that defined tanycyte subpopulations have different neural precursor characteristics: GLAST −ive β-tanycytes are unable to form neurospheres, while GLAST +ive α-tanycytes are neurosphere-forming. Of these, only the dorsal α2 subset have the unlimited self-renewal capacity of stem cells; other subsets appear to represent progenitors with a more limited self-renewal capacity. Finally, through infusion of fibroblast growth factor (FGF)-2 in vivo and inhibition of FGF signalling ex vivo , we demonstrate that FGF signalling is necessary and sufficient for α-tanycyte proliferation. Our study raises the intriguing possibility that local FGF signalling governs cellular homeostasis within a hypothalamic stem cell niche. Distinct tanycyte subpopulations line the third ventricle We first confirmed the location of hypothalamic tanycytes, examining expression of the intermediate filament marker, Vimentin. Expression is restricted to tanycytes ( Fig. 1a ) in the central/posterior hypothalamus ( Supplementary Fig. S1a ) and reveals their cardinal morphological features: a cell body located in the ventricular lining, and a long basally projecting process ( Fig. 1a , right-hand panels) that distinguishes them from ependymocytes. The position and projection of the Vimentin +ive process defines classic tanycyte subsets: β-tanycytes line the median eminence; α2-tanycytes reside adjacent to the arcuate nucleus; α1-tanycytes extend from the level of the ventromedial nucleus to the dorso-medial nucleus ( Fig. 1 ) [25] , [26] . Tanycytes express proteins associated with NSCs in other brain regions: all tanycytes appear to co-express Vimentin and Nestin ( Fig. 1b ) and many appear to express SOXB1 proteins ( Supplementary Fig. S1a,b ) [7] . 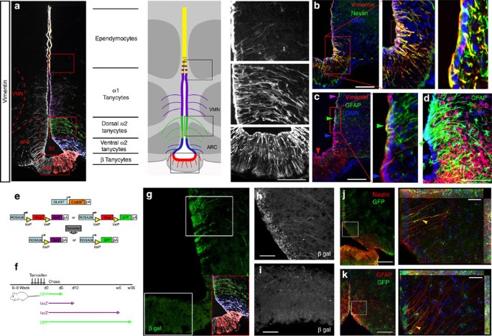Figure 1:GLAST::CreERT2marks α-tanycytes subpopulations in the adult hypothalamus. (a) Left hand panel: coronal section (c.s.) through third ventricle (3V), immunolabelled with Vimentin. The Vimentin+iveprocess distinguishes tanycytes (false-coloured in right-hand side of image) from ependymocytes. Central panel cartoon shows position and process projection of tanycyte subtypes: purple, α1; green, dα2; blue, vα2; red, β. Note β-tanycytes divide into medial β2 and lateral β1 subsets13,14. Right-hand (rh) panel shows high-power magnifications of boxed regions. Ventrally, all ventricular cells appear to have a Vimentin+iveprocess; medially, many ventricular cells have a Vimentin+iveprocess; dorsally, the ependymocyte/α1 boundary is indistinct, with intermingling of tanycytes and ependymocytes. (b–d): Confocal images, showing c.s. through central hypothalamus, counter-stained with DAPI. (b) Double-labelling shows co-expression of Nestin/Vimentin in tanycytes. High-power views (rh panels) show co-expression in most cells. (c) Double-label analysis of Vimentin/GFAP reveals that dα2-tanycytes (boxed, green arrowhead) and some α1-tanycytes (purple arrowhead) but not vα2- (blue arrowheads) or β-tanycytes (red arrowhead) co-express Vimentin/GFAP. (d) Co-labelling with GFAP and Hu reveals long-process dα2-tanycytes (green arrowhead), short-process α1-tanycytes (purple arrowhead) and GFAP−ivevα2-tanycytes (blue arrowhead). (e,f): Schematics, showing (e)GLAST::CreERT2mice27crossed toR26Rmice. Recombination was induced with tamoxifen. Cre-recombinase expressed under GLAST promoter is translocated to nucleus where it floxes a neo cassette, leading to either lacZ expression and βgal production, or to GFP expression, under control of the ubiquitous ROSA26 promoter. (f) Mice were analysed acutely (5 or 10 days) or after longer-term chase periods (6 weeks, 9 months). (g–i):GLAST::CreERT2mice express the reporter, β-gal, in α-tanycytes. Inset ingshows pseuodocoloured regions as in (a). High-power views (taken from regions equivalent to those boxed in (g) show expression in α2-tanycytes (h) but not β-tanycytes (i). (j,k): Double or triple labelling of GFP, Nestin and DAPI (j) or GFP, GFAP and DAPI (k). Yellow arrowheads show GFP expression in dα2-tanycytes. Right-hand panels show high-power views of boxed regions. VMN, ventromedial nucleus; ARC, arcuate nucleus; ME, median eminence. Scale bars:100 μm (a–d,j,k); 20 μm (h,i, rh panels inj,k). Figure 1: GLAST::CreER T2 marks α-tanycytes subpopulations in the adult hypothalamus. ( a ) Left hand panel: coronal section (c.s.) through third ventricle (3V), immunolabelled with Vimentin. The Vimentin +ive process distinguishes tanycytes (false-coloured in right-hand side of image) from ependymocytes. Central panel cartoon shows position and process projection of tanycyte subtypes: purple, α1; green, dα2; blue, vα2; red, β. Note β-tanycytes divide into medial β2 and lateral β1 subsets [13] , [14] . Right-hand (rh) panel shows high-power magnifications of boxed regions. Ventrally, all ventricular cells appear to have a Vimentin +ive process; medially, many ventricular cells have a Vimentin +ive process; dorsally, the ependymocyte/α1 boundary is indistinct, with intermingling of tanycytes and ependymocytes. ( b – d ): Confocal images, showing c.s. through central hypothalamus, counter-stained with DAPI. ( b ) Double-labelling shows co-expression of Nestin/Vimentin in tanycytes. High-power views (rh panels) show co-expression in most cells. ( c ) Double-label analysis of Vimentin/GFAP reveals that dα2-tanycytes (boxed, green arrowhead) and some α1-tanycytes (purple arrowhead) but not vα2- (blue arrowheads) or β-tanycytes (red arrowhead) co-express Vimentin/GFAP. ( d ) Co-labelling with GFAP and Hu reveals long-process dα2-tanycytes (green arrowhead), short-process α1-tanycytes (purple arrowhead) and GFAP −ive vα2-tanycytes (blue arrowhead). ( e , f ): Schematics, showing ( e ) GLAST::CreER T2 mice [27] crossed to R26R mice. Recombination was induced with tamoxifen. Cre-recombinase expressed under GLAST promoter is translocated to nucleus where it floxes a neo cassette, leading to either lacZ expression and βgal production, or to GFP expression, under control of the ubiquitous ROSA26 promoter. ( f ) Mice were analysed acutely (5 or 10 days) or after longer-term chase periods (6 weeks, 9 months). ( g – i ): GLAST::CreER T2 mice express the reporter, β-gal, in α-tanycytes. Inset in g shows pseuodocoloured regions as in ( a ). High-power views (taken from regions equivalent to those boxed in ( g ) show expression in α2-tanycytes ( h ) but not β-tanycytes ( i ). ( j , k ): Double or triple labelling of GFP, Nestin and DAPI ( j ) or GFP, GFAP and DAPI ( k ). Yellow arrowheads show GFP expression in dα2-tanycytes. Right-hand panels show high-power views of boxed regions. VMN, ventromedial nucleus; ARC, arcuate nucleus; ME, median eminence. Scale bars:100 μm ( a – d , j , k ); 20 μm ( h , i , rh panels in j , k ). Full size image Double-label analyses with Nestin shows expression of GFAP in tanycytes lining the third ventricle ( Fig. 1c ). However, in contrast to Vimentin/Nestin, GFAP is restricted to particular tanycyte subsets. Expression is detected, in particular, on dorsal α2-tanycytes (dα2) and some α1-tanycytes ( Fig. 1c green and purple arrowheads, respectively). Little/no GFAP expression is detected on ventral-most α2-tanycytes (vα2) or β-tanycytes ( Fig. 1c blue and red arrowheads, respectively). Thus, GFAP expression distinguishes dα2-tanycytes from vα2- and β-tanycytes. Together, these observations confirm previous studies showing that tanycytes occupy the ventricular lining of the hypothalamus, confirm that tanycytes express markers indicative of neural stem/progenitor cells and reveal the presence of different tanycyte subsets. GLAST::CreER T2 labels α-tanycytes Although recent studies have focused attention on β2-tanycytes as proliferating progenitors [22] , [23] , earlier studies suggested that α-tanycytes may harbour neural stem/progenitor potential in the adult [6] , [11] . To examine whether adult α-tanycytes possess neural stem/progenitor functions, we searched for an appropriate genetic means to label them. Adult GLAST::CreER T2 mice [27] , [28] were crossed with Cre reporter mice that ubiquitously express either β-gal or GFP ( z/EG mice) following Cre-mediated recombination ( Fig. 1e ) [29] , [30] and examined acutely (after 5 or10 days: Fig. 1f ; n =5 mice for each reporter). Reporter activity was detected in the third ventricle in cells with the archetypal features of tanycytes: ventricular-located cell bodies and basally extending processes ( Fig. 1g ). No reporter activity was detected in control uninduced tissue ( Supplementary Fig. S2 ). Cre-recombinase appeared to be restricted to α-tanycytes ( Fig. 1g ) and was particularly concentrated in α2-tanycytes ( Fig. 1h ; Supplementary Fig. S2 ). No expression was detected in β-tanycytes ( Fig. 1i ; Supplementary Fig. S2 ). Double-label analyses with Nestin confirmed the tanycytic nature of reporter +ive cells ( Fig. 1j ). Similarly, co-labelling with GFAP revealed reporter activity in all three α tanycyte subsets (α1-, dα2- and vα2-tanycytes: Fig. 1k ; Supplementary Fig. S2 ). GFAP +ive subventricular astrocytes, which could be distinguished from tanycytes on the basis of their morphology and location, did not co-express the reporter ( Supplementary Fig. S2 ). Together, these analyses suggest that in cells close to the third ventricle, active Cre-recombinase is restricted to α-tanycytes. High-power saturating analyses of the hypothalamus did reveal the presence of recombined cells, additionally, in the parenchymal regions of acutely analysed reporter mice. A small minority (2±1.4/section; 4%) of recombined parenchymal cells co-expressed GFAP and had astrocytic morphology ( Supplementary Fig. S3 ). The vast majority (96%, n =4) of recombined cells in the parenchymal region were GFAP −ive ( Supplementary Fig. S3a ). These morphologically distinct cells could not be identified as progenitor cells (Nestin, NG2) or neurons (NeuN) ( Supplementary Fig. S3b–d ). α-Tanycytes self-renew and give rise to β1-tanycytes We next determined whether α-tanycytes self-renew, whether newly generated tanycytes increase in number over time, and whether α-tanycytes give rise to other (β)-tanycyte subsets. LacZ reporter expression was examined in GLAST::CreER T2 mice acutely and after a series of chase intervals ( n =3 mice each), and the number and extent of labelled tancytes were examined in α2 and β zones. α2-tancyte numbers increased significantly in 6-week-chased animals, these numbers remained constant at 9 months ( Fig. 2a–c ). Intriguingly, labelled tanycytes appeared in zones harbouring β-tanycytes, with the highest numbers detected after a 6-week chase ( Fig. 2a–c ). Labelled tanycytes were consistently detected in the infundibular recess, a region harbouring β1-tanycytes ( Fig. 2b , closed red arrowheads). None was detected in medial-most parts of the median eminence (open red arrowheads). 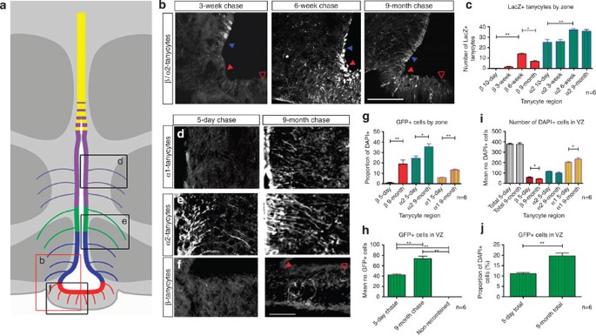Figure 2: Tanycytes expandin vivoin the absence of stimulation. (a) Cartoon indicating regions shown in (b,d,e,f). (b) High-power views of coronal sections through central hypothalamus ofGLAST:CreERT2mice (lacZ reporter) analysed after a 3-week, 6-week or 9-month chase. Lineage-labelled α-tanycytes increase over time (blue arrowhead points to ventral-most boundary of vα2-tanycytes). In addition, lineage-labelled tanycytes increase in the region of the infundibular recess (red closed arrowheads). Red open arrowheads point to the middle of median eminence. Scale bar: 100 μm. (c) Quantitative analyses showing numbers of lacZ+ivetanycytes.n=3 mice each. Unpairedt-test was used to calculateP-values, *,** indicateP<0.05,P<0.01, respectively, error bars represent s.e.m. (d–f) High-power views of coronal sections through central hypothalamus ofGLAST:CreERT2mice (GFP reporter) analysed after a 5-day (left hand panels) or 9-month chase (right-hand panels). Panels show regions containing α1-, α2- and β-tanycytes. Red closed arrowhead points to infundibular recess, red open arrowhead points to median eminence. Scale bar: 50 μm. (g–j) Quantitative analyses of GFP reporter mice reveal a significant increase in the mean proportion of β- α2- and α1-reporter+ivetanycytes (g), and a significant increase in the mean number and proportion of reporter cells located in the VZ (h,j). The mean total number of VZ cells does not significantly alter (i).n=3 mice each. Unpairedt-test was used to calculatePvalues, *,** indicateP<0.05,P<0.01, respectively, error bars represent s.e.m. Figure 2: Tanycytes expand in vivo in the absence of stimulation. ( a ) Cartoon indicating regions shown in ( b , d , e , f ). ( b ) High-power views of coronal sections through central hypothalamus of GLAST:CreER T2 mice (lacZ reporter) analysed after a 3-week, 6-week or 9-month chase. Lineage-labelled α-tanycytes increase over time (blue arrowhead points to ventral-most boundary of vα2-tanycytes). In addition, lineage-labelled tanycytes increase in the region of the infundibular recess (red closed arrowheads). Red open arrowheads point to the middle of median eminence. Scale bar: 100 μm. ( c ) Quantitative analyses showing numbers of lacZ +ive tanycytes. n =3 mice each. Unpaired t -test was used to calculate P -values, *,** indicate P <0.05, P <0.01, respectively, error bars represent s.e.m. ( d – f ) High-power views of coronal sections through central hypothalamus of GLAST:CreER T2 mice (GFP reporter) analysed after a 5-day (left hand panels) or 9-month chase (right-hand panels). Panels show regions containing α1-, α2- and β-tanycytes. Red closed arrowhead points to infundibular recess, red open arrowhead points to median eminence. Scale bar: 50 μm. ( g – j ) Quantitative analyses of GFP reporter mice reveal a significant increase in the mean proportion of β- α2- and α1-reporter +ive tanycytes ( g ), and a significant increase in the mean number and proportion of reporter cells located in the VZ ( h , j ). The mean total number of VZ cells does not significantly alter ( i ). n =3 mice each. Unpaired t -test was used to calculate P values, *,** indicate P <0.05, P <0.01, respectively, error bars represent s.e.m. Full size image Analysis of GFP-reporter GLAST::CreER T2 mice revealed a similar pattern. Here, the extent and density of labelled tanycytes was quantified in three zones, harbouring β-tanycytes, α2-tanycytes and α1-tanycytes/ependymal cells in acute-culled (5 days post-recombination) versus 9-month-chased mice (schematic Fig. 2a ; n =3 mice each). These analyses revealed a significant increase in extent and density of reporter +ive tanycytes at 9 months compared with that at 5 days in all three zones ( Fig. 2d–h ). No difference was observed in the total number of VZ cells over this period ( Fig. 2i ), indicating that they must be replaced over time. These results suggest that tanycytes proliferate in the adult mouse and indicate that their progeny can self-renew to give rise to more α2-tanycytes, or can give rise to more ventral, or more dorsal tanycytes that lie in domains harbouring β1- and dorsal α1-tanycytes, respectively. GLAST::CreER T2 cells are gliogenic and neurogenic We next determined whether the progeny of GLAST::CreER T2 cells give rise to glia and neurons, analysing reporter-positive cells in the central hypothalamus of 6-week- and 9-month-chased mice in comparison to acute-culled animals. These analyses revealed a significant increase in reporter +ive GFAP +ive astrocytes located in non-ventricular regions ( Fig. 3a–d ; Supplementary Fig. S4a,b ). Six weeks post recombination, newly generated reporter +ive GFAP +ive cells appeared restricted to sub-/periventricular regions ( Fig. 3a , yellow arrows; Supplementary Fig. S4a ) and were associated with tanycyte processes ( Fig. 3b , red arrow 2). Reporter activity was not detected in GFAP +ive cells in parenchymal regions ( Fig. 3a , arrow 4; Supplementary Fig. S4a ). By contrast, after a 9-month chase reporter +ive /GFAP +ive cells were detected in parenchymal regions ( Fig. 3c , yellow arrows) and were located particularly in ventral regions around the arcuate and ventromedial nuclei ( Supplementary Fig. S4a ). Of the reporter +ive cells analysed after a 9-month chase, 44% differentiated into astrocytes ( Supplementary Fig. S4d ), constituting the majority of the non-ventricular reporter +ive cells. 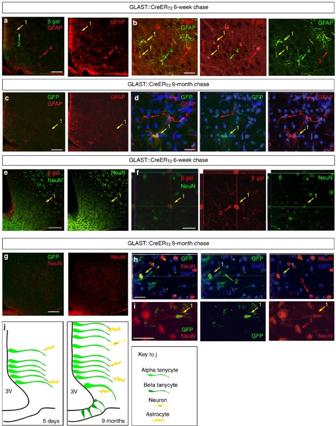Figure 3:GLAST::CreERT2cells are gliogenic and neurogenic. (a–i) Coronal sections ofGLAST::CreERT2mice after 6-week (a,b,e,f; β-gal reporter) or 9-month chase (c,d,g–i; GFP reporter). Images show single-, dual- and triple-channel views after immunolabelling to detect reporter activity, DAPI and GFAP (a–d) or reporter activity, DAPI and NeuN (e–i). (a,b): Low-power (a) or high-power confocal (b) views. After 6-week chase, GFP+iveGFAP+ivecells with astrocyte morphology are detected in periventricular regions (yellow arrows, 1) and associated with reporter-positive tanycytes (arrows, 2), rather than with reporter-positive parenchymal cells (arrows, 3). GFAP+ivecells in lateral parenchymal regions (arrows, 4) do not co-express the reporter. (c,d): Low-power (c) or high-power confocal (d) views. After 9-month chase, GFAP+iveGFP+iveastrocytes (yellow arrows, 1) intermingle with GFAP+ivereporter-iveastrocytes (red arrows, 2) in lateral parenchymal regions. (e,f): Low-power (e) or high-power confocal (f) views. Yellow arrows (1) point to NeuN+iveβ-gal+ivecell, outside the VMN, and closely associated with β-gal+ivetanycyte process (red arrow, 2). Although many NeuN+ivecells are detected in the VMN, none expresses the reporter. (g–i): Low (g) or high-power (h,i) views. After 9-month chase, NeuN+iveGFP+ivecells are detected (yellow arrows, 1). Panel (h) shows neuronal cell close to the SVZ and closely associated with a reporter+ivetancyte process (green arrow, 2). Panel (i) shows reporter+iveneuronal cell (yellow arrow, 1) in VMN. In (h,i), red arrows (3) show reporter-iveNeuN+iveneurons. (j) Schematic summarising lineage-tracing analyses. At 5 days after recombination, reporter activity is concentrated in α2-tanycyte populations. After 9-month chase, increased numbers of reporter+ivecells are detected in α2 region, and in dorsal (α1/ependyma) and ventral (β1) regions. Scale bars: 100 μm (a,c,e,g); 20 μm (b,d,f,h,i). Figure 3: GLAST::CreER T2 cells are gliogenic and neurogenic. ( a – i ) Coronal sections of GLAST::CreER T2 mice after 6-week ( a , b , e , f ; β-gal reporter) or 9-month chase ( c , d , g – i ; GFP reporter). Images show single-, dual- and triple-channel views after immunolabelling to detect reporter activity, DAPI and GFAP ( a – d ) or reporter activity, DAPI and NeuN ( e–i ). ( a , b ): Low-power ( a ) or high-power confocal ( b ) views. After 6-week chase, GFP +ive GFAP +ive cells with astrocyte morphology are detected in periventricular regions (yellow arrows, 1) and associated with reporter-positive tanycytes (arrows, 2), rather than with reporter-positive parenchymal cells (arrows, 3). GFAP +ive cells in lateral parenchymal regions (arrows, 4) do not co-express the reporter. ( c , d ): Low-power ( c ) or high-power confocal ( d ) views. After 9-month chase, GFAP +ive GFP +ive astrocytes (yellow arrows, 1) intermingle with GFAP +ive reporter -ive astrocytes (red arrows, 2) in lateral parenchymal regions. ( e , f ): Low-power ( e ) or high-power confocal ( f ) views. Yellow arrows (1) point to NeuN +ive β-gal +ive cell, outside the VMN, and closely associated with β-gal +ive tanycyte process (red arrow, 2). Although many NeuN +ive cells are detected in the VMN, none expresses the reporter. ( g – i ): Low ( g ) or high-power ( h , i ) views. After 9-month chase, NeuN +ive GFP +ive cells are detected (yellow arrows, 1). Panel ( h ) shows neuronal cell close to the SVZ and closely associated with a reporter +ive tancyte process (green arrow, 2). Panel ( i ) shows reporter +ive neuronal cell (yellow arrow, 1) in VMN. In ( h , i ), red arrows (3) show reporter -ive NeuN +ive neurons. ( j ) Schematic summarising lineage-tracing analyses. At 5 days after recombination, reporter activity is concentrated in α2-tanycyte populations. After 9-month chase, increased numbers of reporter +ive cells are detected in α2 region, and in dorsal (α1/ependyma) and ventral (β1) regions. Scale bars: 100 μm ( a , c , e , g ); 20 μm ( b , d , f , h , i ). Full size image In contrast to the abundant de novo -generated astrocytes, very small, albeit significant, numbers of reporter +ive NeuN +ive neurons were generated ( Fig. 3e–i ) over a 9-month period. In 6-week-chased animals, reporter +ive NeuN +ive cells were never observed within a defined hypothalamic nucleus, but instead were closely associated with tanycytic processes in the periventricular region ( Fig. 3e ; Supplementary Fig. S4c ). In 9-month-chased animals, ~50% reporter +ive NeuN +ive cells were similarly closely associated with tanycyte processes in the sub-/periventricular zone ( Fig. 3h ; Supplementary Fig. S4c ). The remaining NeuN +ive cells were observed in, and close to, the arcuate and ventromedial nuclei ( Fig. 3i ; Supplementary Fig. S4c ). In total, at 6 weeks and 9 months, NeuN +ive cells constituted 1–2% of reporter +ive cells ( Supplementary Fig. S4d ). At both 6 weeks and 9 months, many of the remaining periventricular/parenchymal reporter +ive cells were closely associated with tanycyte processes. To ask whether these might be neuronal precursors that are generated in abundance, but are eliminated or migrate away, we examined their expression of doublecortin, a marker of neuronal progenitors. Doublecortin +ive reporter +ive cells were not detected in acute-culled GLAST::CreER T2 mice, but were detected after a 6-week chase ( Supplementary Fig. S4e–g ). However, they were sparse in number, constituting only 5% of reporter +ive cells ( Supplementary Fig. S4h ). This, together with their unusual astrocytic morphology ( Supplementary Fig. S4i ), does not support the idea that high numbers of neuronal progenitors are generated in the unchallenged mouse. We conclude that GLAST +ive α-tanycytes include neural stem/progenitor population(s) that can proliferate and differentiate into astrocytic and neuronal lineages (schematic Fig. 3j ), albeit realising their neurogenic potential at extremely low levels under normal conditions. α-Tanycytes proliferate in response to FGF-2 in vivo In both the SVZ and the SGZ, NSCs actively respond to FGF-2 by increasing their proliferation and survival, both in vivo and in vitro [31] . Therefore, we next ascertained whether α-tanycytes are FGF-responsive in vivo . BrdU, or BrdU and FGF-2 were infused intracerebroventricularly into adult mice for 7 days, and the mice were killed either immediately or 6 weeks post infusion ( Fig. 4 , top schematic, n =4 mice each). 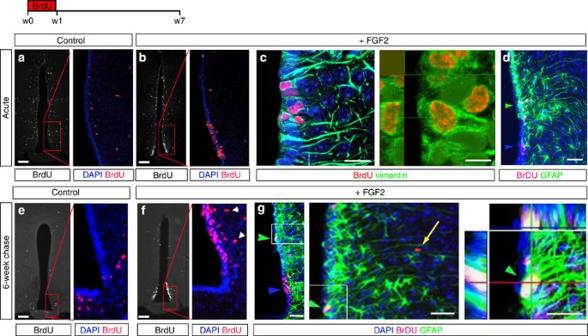Figure 4: α-Tanycytes are FGF-responsive progenitorsin vivo. Cartoon: schematic showing infusion and chase regimes in weeks (w). (a–d): Coronal sections through central hypothalamus of mice infused with BrdU (a) or BrdU and FGF-2 (b–d) for 1 week and killed immediately. Right-hand panels ina,b,cshow high-power views. Double-labelling with vimentin (c) indicates that newborn α2-tanycytes retain their identity. Double-labelling with GFAP (d) distinguishes vα2/dα2-tanycyctes: both dα2 (green arrowheads) and vα2 (blue arrowheads) subtypes show increase in BrdU-labelling. (e–g)Coronal sections through central hypothalamus of mice infused with BrdU alone (e) or with FGF-2 (f,g) for 1 week, and killed 6 weeks later. Right-hand panels ine,f,gshow high-power views of boxed regions. Ventricular and periventricular (white arrowheads) cells in the region of α-tanycytes proliferate after FGF-2 exposure (f). Some BrdU+ivecells are detected in parenchymal regions, closely associated with tanycyte processes (g, yellow arrow in middle panel). Confocal microscopy reveals a BrdU+ivedα2-tanycyte that co-expresses GFAP (green arrowhead ing, middle and right-hand panels). Scale bars: 100 μm (a,b,e,f; high-power views 30 μm); 50 μm (d,gleft panel); 30 μm (cleft-hand panel,gmiddle panel); 20 μm (g, right panel); 10 μm (c′). Figure 4: α- Tanycytes are FGF-responsive progenitors in vivo . Cartoon: schematic showing infusion and chase regimes in weeks (w). ( a – d ): Coronal sections through central hypothalamus of mice infused with BrdU ( a ) or BrdU and FGF-2 ( b – d ) for 1 week and killed immediately. Right-hand panels in a , b , c show high-power views. Double-labelling with vimentin ( c ) indicates that newborn α2-tanycytes retain their identity. Double-labelling with GFAP ( d ) distinguishes vα2/dα2-tanycyctes: both dα2 (green arrowheads) and vα2 (blue arrowheads) subtypes show increase in BrdU-labelling. ( e – g) Coronal sections through central hypothalamus of mice infused with BrdU alone ( e ) or with FGF-2 ( f , g ) for 1 week, and killed 6 weeks later. Right-hand panels in e , f , g show high-power views of boxed regions. Ventricular and periventricular (white arrowheads) cells in the region of α-tanycytes proliferate after FGF-2 exposure ( f ). Some BrdU +ive cells are detected in parenchymal regions, closely associated with tanycyte processes ( g , yellow arrow in middle panel). Confocal microscopy reveals a BrdU +ive dα2-tanycyte that co-expresses GFAP (green arrowhead in g , middle and right-hand panels). Scale bars: 100 μm ( a , b , e , f ; high-power views 30 μm); 50 μm ( d , g left panel); 30 μm ( c left-hand panel, g middle panel); 20 μm ( g , right panel); 10 μm ( c ′). Full size image FGF-2 infusion significantly enhanced proliferation in hypothalamic VZ cells ( P =0.0078), but did not enhance acute proliferation within either the subventricular region ( P =0.53) or median eminence cells ( P =0.53) in immediately killed animals ( Fig. 4a ; Supplementary Fig. S5a ). To examine the character of BrdU +ive VZ cells, we performed double-label analyses with Vimentin. These analyses confirmed that Vimentin +ive tanycytes proliferate in response to FGF-2 ( Fig. 4c ). Double-labelling with GFAP, to distinguish the response of different tanycyte subsets ( Fig. 1 ), revealed that α2-tanycytes exhibit the highest response: a 51-fold increase ( P =0.0015) in BrdU-labelling in vα2-tanycytes and a 6-fold increase ( P =0.023) in dα2-tanycytes ( Fig. 4d , blue and green arrowheads, respectively; Supplementary Fig. S5b ). By contrast, there was no increase in BrdU incorporation into regions of the ventricle containing β-tanycytes ( P =0.097) and no significant increase ( P =0.17) in BrdU incorporation into regions occupied by α1-tanycytes ( Fig. 4b , Supplementary Fig. S5b ). After a longer-term (6-week) chase, FGF-2 treatment still resulted in a significant increase ( P =0.007) in label-retaining cells in the ventricular region ( Fig. 4e ; Supplementary Fig. S5c ). Additionally, a significant increase (five-fold, P =0.004) in BrdU-labelled cells was now detected in the sub-/periventricular region (arrowheads in Fig. 4f ), with no change within the median eminence ( Fig. 4f ; Supplementary Fig. S5c ). Co-labelling with GFAP revealed particularly abundant numbers of BrdU-labelled vα2- ( Fig. 4g , blue arrowhead, Supplementary Fig. S5d ) and dα2-tanycytes ( Fig. 4g , green arrowhead, Supplementary Fig. S5d ). The temporal progression of BrdU-labelling from tanycytes soon after FGF-infusion to sub-/periventricular cells, 6 weeks later, raises the possibility that tanycytes may be the progenitors of these newborn cells. α-Tanycytes are neurospherogenic To examine whether α-tanycytes respond directly to FGF signalling, we employed the neurosphere assay, which supports expansion of cells with proliferative, stem cell-like potential. Previous studies have suggested that adult hypothalamic cells can form multipotent self-renewing neurospheres [7] , [10] , [11] , [32] , but have not strictly established that tanycytes are neurospherogenic. We first asked whether neurosphere-forming ability is restricted to tanycyte-containing regions. Tanycytes are largely absent from the anterior hypothalamus and from dorsal ventricular regions of the third ventricle [17] , [22] , [33] . Anterior, central and posterior hypothalamic slices were accurately subdissected on the basis of arginine-vasopressin, neuropeptide-Y, Fgf-10 and Fgf-18 expression ( Fig. 5a , top schematic; Fig. 5b ; full profiles shown in Supplementary Fig. S6 ), and each was tested for its ability to generate neurospheres ( n =6). Marked differences were found: the anterior hypothalamus generated very few/no neurospheres that failed to passage; the central hypothalamus generated substantial numbers of neurospheres that could be maintained and expanded (at least to 25 passages: the latest examined); the posterior hypothalamus formed lower numbers of neurospheres that could also be expanded in vitro ( Fig. 5c ). Thus, neurospherogenic potential correlates with tanycyte location along the anterior–posterior axis. 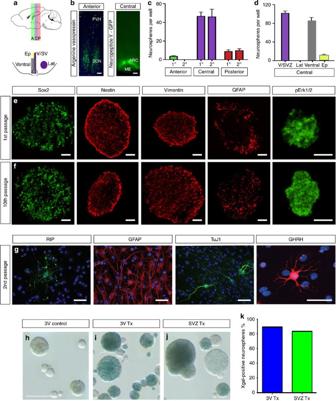Figure 5: Neurospherogenic potential resides in α-tanycytes. (a–d): Different zones of the hypothalamus vary in their ability to form neurospheres. (a) Cartoon illustrating anterior–posterior subdissection (top panel) and mediolateral/dorsoventral subdissections (bottom panel); accuracy of dissection along A–P axis was confirmed on the basis of AVP (anterior-specific) and NPY (central-specific) expression (b). (c) Anterior hypothalamic regions generate no passageable spheres. Large numbers of neurospheres can be derived from the central, and lower numbers from the posterior, hypothalamus (n=6; error bars show s.e.m.). (d): Within the central hypothalamus, neurospherogenic potential lies in the VZ/SVZ, with highest activity in ventral tanycyte-containing regions. Neurospheres formed from VZ/SVZ cells, but not from lateral parenchymal cells (n=6; error bars show s.e.m.). (e,f): Antibody labelling in primary and tenth passage neurospheres. Neurospheres express Sox2, Nestin, Vimentin and pErk1/2 in a high proportion of cells, and GFAP in a subset of cells. (g): Differentiated neurospheres express markers indicative of all three neural lineages. GHRH+ivelabelling indicates formation of hypothalamic neurons. (h–k): Neurospheres derived from the hypothalamus ofGLAST::CreERT2mice express the reporter β-gal (i,l), indicating their descent from tanycytes. Unrecombined mice and recombined lateral ventricle SVZ show negative and positive controls (h,jrespectively). Scale bars:100 μm (b); 50 μm (e,f); 20 μm (g); 250 μm (h). PVH, paraventricular nucleus; SCN, suprachiasmatic nucleus; rest as inFig. 1. Figure 5: Neurospherogenic potential resides in α-tanycytes. ( a – d ): Different zones of the hypothalamus vary in their ability to form neurospheres. ( a ) Cartoon illustrating anterior–posterior subdissection (top panel) and mediolateral/dorsoventral subdissections (bottom panel); accuracy of dissection along A–P axis was confirmed on the basis of AVP (anterior-specific) and NPY (central-specific) expression ( b ). ( c ) Anterior hypothalamic regions generate no passageable spheres. Large numbers of neurospheres can be derived from the central, and lower numbers from the posterior, hypothalamus ( n =6; error bars show s.e.m.). ( d ): Within the central hypothalamus, neurospherogenic potential lies in the VZ/SVZ, with highest activity in ventral tanycyte-containing regions. Neurospheres formed from VZ/SVZ cells, but not from lateral parenchymal cells ( n =6; error bars show s.e.m.). ( e , f ): Antibody labelling in primary and tenth passage neurospheres. Neurospheres express Sox2, Nestin, Vimentin and pErk1/2 in a high proportion of cells, and GFAP in a subset of cells. ( g ): Differentiated neurospheres express markers indicative of all three neural lineages. GHRH +ive labelling indicates formation of hypothalamic neurons. ( h – k ): Neurospheres derived from the hypothalamus of GLAST::CreER T2 mice express the reporter β-gal ( i , l ), indicating their descent from tanycytes. Unrecombined mice and recombined lateral ventricle SVZ show negative and positive controls ( h , j respectively). Scale bars:100 μm ( b ); 50 μm ( e , f ); 20 μm ( g ); 250 μm ( h ). PVH, paraventricular nucleus; SCN, suprachiasmatic nucleus; rest as in Fig. 1 . Full size image We next assayed the neurospherogenic potential of mediolateral and dorsoventral sub-domains within the central hypothalamus (bottom schematic, Fig. 5a ). Neurospheres formed from ventricular/subventricular regions, but not from lateral/parenchymal regions ( Fig. 5d ). Similarly, while neurospheres formed readily from ventral (tanycyte-rich) regions of the ventricular region, the ability of neurospheres to form from dorsal ventricular regions (ependymocyte-rich) was sparse ( Fig. 5d ). These results show that neurospherogenic potential correlates with tanycte location. Neurospheres from the central hypothalamus (tissue subdissected from ventral ventricular/subventricular regions) could be stably propagated: late-passage (passage 10) spheres displayed an identical expression profile for the neural stem/progenitor markers, Sox2, Nestin, Vimentin, GFAP, and pErk1/2, an indicator of growth-factor response, compared with primary spheres ( Fig. 5e ). Both early- and late-passage neurospheres differentiated after growth factor reduction, as assessed by the presence of RIP +ive oligodendrocytes [34] , GFAP + cells with astrocytic morphology [35] , TUJ1 +ve immature neurons [36] , [37] and growth hormone releasing hormone (GHRH) +ive hypothalamic neurons [32] ( Fig. 5g ). To prove that neurospherogenic potential resides in α-tanycytes, we asked whether we could derive neurospheres from the third ventricle lining of GLAST::CreER T2 R26R mice, or, as a control, the SVZ of the lateral ventricle. Similar numbers of neurospheres were generated from reporter mice and wild-type mice (91±7 spheres per well; compare with Fig. 5d ). Moreover, X-gal staining revealed that the majority of third ventricle-derived neurospheres (89%) arose from recombined progenitors, comparable to the proportion of recombined progenitors formed from the SVZ (83%) ( Fig. 5h–k ). Together, these analyses show that α-tanycytes are neurospherogenic. Self-renewing neurospheres correlate with dα2-tanycytes In situ hybridisation analyses reveal that Fgf-10 and Fgf-18 are specifically detected in the adult hypothalamus. Both are detected in the central/posterior hypothalamus, but not in the anterior hypothalamus ( Fig. 6a ; Supplementary Figs S6 and S7 , see also ref. 12 ). High levels of Fgf-10 are detected in the territory occupied by vα2- and β-tancytes, whereas Fgf-18 marks just the region occupied by vα2-tanycytes ( Fig. 6a–d ; Supplementary Fig. S7 ). 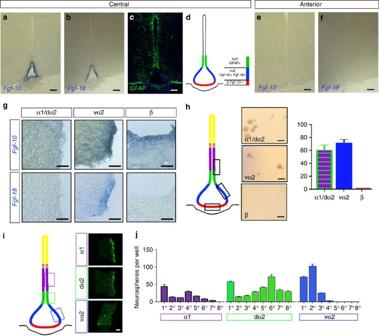Figure 6: Dorsoventral differences in neurosphere formation and maintenance correlate with tanycyte subtypes. (a–d) Expression ofFgf-10,Fgf-18and GFAP in serial adjacent coronal sections through central hypothalamus. Expression profiles correlate with distinct tanycyte subsets (schematic,d). (e,f) NeitherFgf-10norFgf-18are detected in the anterior hypothalamus. (g,h) Tanycyte subtypes differ in neurosphere-forming potential. Subdissections of the hypothalamus (shown schematically inh) allowed β, vα2 and dα2/α1-tanycytes to be cultured separately. Accuracy of dissection was determined through expression ofFgf-10andFgf-18in isolated sister explants (g). β-tanycytes do not form neurospheres whereas vα2 and dα2/α1 regions produce numerous spheres (h;n=6). (i) Further subdissection to separate regions containing vα2, dα2 and α1-tanycytes. Accuracy of dissection was determined in sister explants through expression of GFAP. (j) Neurosphere propagation shows spheres derived from α1-tanycyte-containing regions are not maintained beyond the seventh passage; regions harbouring dα2-tanycytes passage indefinitely; regions harbouring vα2-tanycytes form neurospheres that cannot be maintained beyond the fourth passage (n=2, error bars show s.e.m.). Scale bars: 50 μm (a–f); 30 μm (g); 100 μm (h). Figure 6: Dorsoventral differences in neurosphere formation and maintenance correlate with tanycyte subtypes. ( a – d ) Expression of Fgf-10 , Fgf-18 and GFAP in serial adjacent coronal sections through central hypothalamus. Expression profiles correlate with distinct tanycyte subsets (schematic, d ). ( e , f ) Neither Fgf-10 nor Fgf-18 are detected in the anterior hypothalamus. ( g , h ) Tanycyte subtypes differ in neurosphere-forming potential. Subdissections of the hypothalamus (shown schematically in h ) allowed β, vα2 and dα2/α1-tanycytes to be cultured separately. Accuracy of dissection was determined through expression of Fgf-10 and Fgf-18 in isolated sister explants ( g ). β-tanycytes do not form neurospheres whereas vα2 and dα2/α1 regions produce numerous spheres ( h ; n =6). ( i ) Further subdissection to separate regions containing vα2, dα2 and α1-tanycytes. Accuracy of dissection was determined in sister explants through expression of GFAP. ( j ) Neurosphere propagation shows spheres derived from α1-tanycyte-containing regions are not maintained beyond the seventh passage; regions harbouring dα2-tanycytes passage indefinitely; regions harbouring vα2-tanycytes form neurospheres that cannot be maintained beyond the fourth passage ( n =2, error bars show s.e.m.). Scale bars: 50 μm ( a – f ); 30 μm ( g ); 100 μm (h). Full size image We used these markers to determine whether we could detect any variation in neurospherogenic behaviour in different α-tanycyte subpopulations, refining the subdissections of central hypothalamic slices, to separate ventricular regions containing Fgf-10 −ive /Fgf-18 −ive α1/dα2-tanycytes, Fgf-10 +ive /Fgf-18 +ive vα2-tanycytes and, as controls, Fgf-10 +ive /Fgf-18 −ive β-tanycytes ( Fig. 6g , cartoon). Identical explants were then dissociated, and cells from each region examined for neurospherogenic behaviour. Marked differences were detected in the neurosphere-generating ability of α- or β-tanycyte-containing regions. Robust numbers of neurospheres could be generated from cells derived from either dα2/α1- or vα2-tanycytes. By contrast, no neurospheres could be derived from subdissections containing only β-tanycytes ( Fig. 6h ). Although equivalent numbers of neurospheres formed from regions containing either dα2/α1- and vα2-tanycytes, propagation of these neurosphere subsets revealed subtly different behaviours. Further subdissection of regions harbouring α1- or dα2-tanycytes showed that only regions containing dα2-tanycytes (defined through GFAP on long processes; Fig. 6i ) showed stem-like characteristics, generating neurospheres that self-renewed robustly, consistently producing stable numbers of neurospheres that could be passaged extensively (at least 25 passages; the latest examined; Fig. 6j ). By contrast, although regions harbouring GFAP -ive / Fgf-10 +ive /Fgf-18 +ive vα2-tanycytes ( Fig. 6g ) proliferated readily, generating large numbers of primary spheres, these had a limited self-renewal capacity, failing to propagate beyond the 4th passage ( Fig. 6j ). Similarly, regions containing α1-tanyctes (defined through sporadic GFAP on short processes; Fig. 6i ) formed neurospheres, but these failed to propagate beyond the 7th passage ( Fig. 6j ). FGF signalling is required for α2-tancycyte proliferation To directly test the requirement of hypothalamic neurospheres for FGF, primary hypothalamic cell suspensions were cultured in the absence of FGF-2, or, for comparison, the absence of EGF or both ( Fig. 7a ). Exogenous EGF and FGF were required for the formation of 70% of neurospheres. FGF was required for sphere formation by ~40% of the primary neurospheres, whereas most primary neurospheres (~90%) formed in the absence of EGF. These data suggest that EGF and FGF do not have a synergistic effect on primary sphere formation, and instead suggest that, during primary neurosphere formation, FGF>EGF as a mitogen for NSCs and/or progenitors. By contrast, both EGF and FGF appeared to be required for the maintenance of neurospheres: 90% neurospheres required FGF to support their propagation and 100% showed a complete dependence on exogenous EGF ( Fig. 7a ). 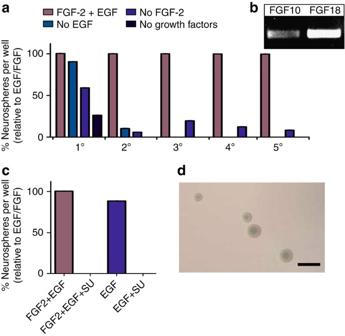Figure 7: Hypothalamic neurospheres are FGF-responsive. (a) Primary neurospheres grown in the presence or absence of FGF-2 and EGF. Addition of both factors produces consistently high numbers of neurospheres over five passages. Without EGF, neurospheres fail to passage; without FGF-2, low numbers of spheres can be maintained for five passages (n=3). (b) Primary neurospheres expressFgf-10andFgf18mRNAS (427 and 438 nucleotides, respectively). (c) Addition of SU5402 to primary neurospheres grown in either FGF-2+EGF or EGF alone prevents neurosphere formation. (d) When hypothalamic cells are spun out of FGF+EGF+SU5402 after 10 days in culture, and replated in fresh FGF+EGF medium, new neurospheres are observed 10 days later. Scale bar: 100 μm. Figure 7: Hypothalamic neurospheres are FGF-responsive. ( a ) Primary neurospheres grown in the presence or absence of FGF-2 and EGF. Addition of both factors produces consistently high numbers of neurospheres over five passages. Without EGF, neurospheres fail to passage; without FGF-2, low numbers of spheres can be maintained for five passages ( n =3). ( b ) Primary neurospheres express Fgf-10 and Fgf18 mRNAS (427 and 438 nucleotides, respectively). ( c ) Addition of SU5402 to primary neurospheres grown in either FGF-2+EGF or EGF alone prevents neurosphere formation. ( d ) When hypothalamic cells are spun out of FGF+EGF+SU5402 after 10 days in culture, and replated in fresh FGF+EGF medium, new neurospheres are observed 10 days later. Scale bar: 100 μm. Full size image The observation that FGFs are expressed within tanycyte-containing regions ( Fig. 6a ), potentially in tanycytes themselves ( Supplementary Fig. S7 ) [23] , raises the possibility that the small numbers of spheres that can be propagated without exogenous FGF produce endogenous FGFs, negating the need for an external source. Analysis of Fgf-10 and Fgf-18 expression in hypothalamic neurospheres revealed that both transcripts are indeed detected ( Fig. 7b ; Supplementary Fig. S8 ). We therefore cultured neurospheres derived from primary hypothalamic cell suspensions in the presence of the FGF signalling inhibitor SU5402 in medium supplemented with both FGF-2 and EGF, or EGF alone. SU5402 abrogated neurosphere formation even in medium containing EGF alone ( Fig. 7c ). To exclude a non-specific toxic effect of the inhibitor, cells from the FGF-2/EGF/SU5402-treated cultures were replated in FGF-2/EGF-supplemented medium. After 10 days, large neurospheres were observed ( Fig. 7d ). Together, this shows the endogenous production of an FGF signal, upon which hypothalamic spherogenic cells depend. Finally, to directly test whether endogenous FGFs are required for the proliferation of α2-tanycytes, hypothalamic slices were cultured ex vivo , alone or with FGF-2, both with and without SU5402. The basic pattern of proliferation detected in vivo using the mitotic marker PH3 was maintained ex vivo , with FGF-2 stimulating a significant increase in proliferation in Nestin +ive α2-tanycytes ( Fig. 8a ). By contrast, FGF signal inhibition significantly reduced Nestin +ive α2-tanycyte proliferation ( Fig. 8b ). These results, together with our in vivo data, support the conclusion that neural stem and progenitor potential resides in subpopulations of α-tanycytes, which can proliferate and differentiate, primarily into astrocytic lineages under normal conditions, and whose proliferation is responsive to local FGF ligands. 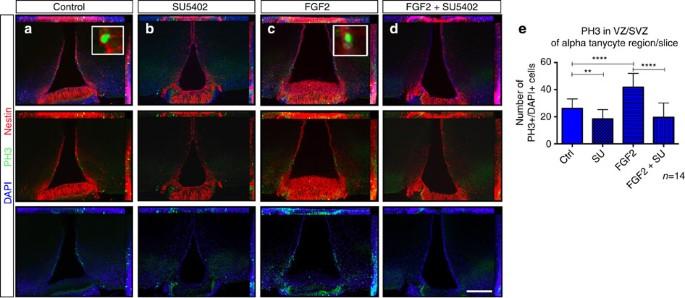Figure 8: Endogenous FGFs govern α-tanycyte proliferationex vivo. (a–d) Whole-mount immunohistochemical analyses of slice cultures of central hypothalamus, cultured alone (a), with SU5402 (b), FGF-2 (c) or FGF-2 and SU5402 (d). Insets in (a,c) show high-power views, showing PH3 expression in Nestin+ivetanycytes. (e): Quantitative analyses shows that FGF-2 stimulates a significant increase in proliferation.n=14. Unpairedt-test was used to calculateP-values, ** and *** indicateP<0.05 andP<0.0001, respectively, and error bars represent s.e.m. Thickness of slices precluded clear identification of precise location (VZ or SVZ) of all PH3+ivecells. Scale bar: 100 μm. Figure 8: Endogenous FGFs govern α-tanycyte proliferation ex vivo . ( a – d ) Whole-mount immunohistochemical analyses of slice cultures of central hypothalamus, cultured alone ( a ), with SU5402 ( b ), FGF-2 ( c ) or FGF-2 and SU5402 ( d ). Insets in ( a , c ) show high-power views, showing PH3 expression in Nestin +ive tanycytes. ( e ): Quantitative analyses shows that FGF-2 stimulates a significant increase in proliferation. n =14. Unpaired t -test was used to calculate P -values, ** and *** indicate P <0.05 and P <0.0001, respectively, and error bars represent s.e.m. Thickness of slices precluded clear identification of precise location (VZ or SVZ) of all PH3 +ive cells. Scale bar: 100 μm. Full size image Our studies provide evidence that hypothalamic α-tanycytes are neural stem and progenitor-like cells. In the unchallenged adult mouse, α-tanycytes can self-renew, or give rise to β-tanycytes and parenchymal astrocytes, and even generate sparse numbers of neurons. FGF signalling appears to have a critical role in cellular homeostasis within the adult hypothalamus, required to promote the proliferation of α-tanycytes. The localised expression of FGF ligands in and adjacent to the niche suggests that α-tanycytes are sensitive to local endogenous signals. A number of lines of evidence support these conclusions. First, only hypothalamic cells from α-tanycyte-rich regions display the archetypal features of NSCs, generating self-renewing multipotent neurospheres in vitro under standard conditions. Importantly, reporter-expressing cells from GLAST::CreER T2 mice are similarly neurospherogenic. As GLAST::CreER T2 mice express active Cre-recombinase in α-tanycytes, but not in subependymal astrocytes or β-tanycytes, this suggests that, within ventricular hypothalamic regions, α-tanycyctes can self-renew. Lineage-tracing studies of the GLAST::CreER T2 mice provide compelling supportive evidence that tanycytes proliferate in vivo under basal conditions, giving rise primarily to additional tanycytes, including β-tanycytes, and to GFAP +ive parenchymal cells, and to very small numbers of neurons that persist long-term and are associated with hypothalamic nuclei. As GLAST::CreER T2 mice express the reporter in unidentified (GFAP −ive NG2 −ive Nestin −ive ) cells within parenchymal regions, there remains the possibility that these cells contribute to de novo generation of adult cells. However, in short-term (3–6-week) chase experiments, newly generated GLAST +ive cells are restricted to ventricular/subventricular regions, or are associated with tanycyte processes, while GLAST +ive cells decline in number in parenchymal regions, supporting the idea that new cells derive from tanycytic, not parenchymal, GLAST +ive cells. Together, these findings support previous fate-mapping data [11] , and strongly suggest that hypothalamic α-tanycytes are adult neural stem and progenitor cells. Our analyses reveal that tanycyte subpopulations can be defined on the basis of characteristic molecular signatures that correlate with a distinctive behaviour of each subpopulation ( Table 1 ). Our in vitro data reveal that only α-tanycytes, and not β2-tanycytes, are FGF-responsive and neurospherogenic (note that our subdissection precluded β1-tanycyte analysis). α1, ventral and dorsal α2-tanycyte subpopulations each proliferate in response to FGF-2 signalling in vivo , but only dorsal α2-tanycytes display the hallmarks of NSCs. They form neurospheres with unlimited self-renewal (up to 25 passages), which are multipotent. By contrast, α1- and ventral α2-tanycytes lack unlimited self-renewal capacity. Our in vivo analyses corroborate these findings, demonstrating that α-tanycytes can self-renew or give rise to more ventrally located β-tanycytes. Lineage-marked β-tanycytes populate the infundibular recess and decline over time, suggesting that α2-tanycytes give rise to progenitor-like β1-tanycytes, potentially including Fgf-10 +ive ventral tanycytes that can give rise to arcuate neurons [23] . However, we find no evidence that α2-tancytes give rise to β2-tanycytes, suggesting a very different origin of these two populations. In summary, α2-tanycytes appear to be infrequently dividing stem-like cells that give rise to cells with limited renewal potential. Table 1 Characteristics of hypothalamic ventricular cells. Full size table Our findings contrast with a recent lineage-tracing study, showing that β2-tanycytes proliferate and generate large numbers of neurons in the median eminence of the postnatal/juvenile hypothalamus [22] , indicative of β2-tanycytes having NSC potential. Notwithstanding differences in ages (juvenile versus adult) and regimes (high-fat diet versus unchallenged), we find that β2-tanycytes are neither FGF-responsive, nor neurospherogenic under standard conditions. These findings indicate, instead, that tanycyte subsets are functionally distinct in terms of NSC potential, and that α2 and β2 subsets respond to different stimuli. Previous studies show that different tanycyte subsets exhibit different functions [5] , and the notion that α2 and β2 subsets could be functionally distinct NSCs may explain why compromised function of each results in very different effects on body weight in response to high-fat diet [7] , [13] , [22] . Hypothalamic tanycytes resemble the NSC of the lateral ventricle, the type B1 astrocyte. Both have a soma located near the ventricle and a long elongated projection to a blood vessel [38] , [39] , [40] , [41] ; both are thought to derive from embryonic radial glia [5] , [14] , [42] ; both express Nestin and divide infrequently. Intriguingly, in the unchallenged mouse, α-tanycytes do not share the highly active neurogenic properties of the type B1 astrocyte, but instead are gliogenic (this paper; also see Wang et al. [5] ). Our recent demonstration that high-fat diet causes expansion of neurosphere-forming ventricular cells [43] , together with the data presented here, suggests that α-tanycyte behaviour is under robust physiological and environmental regulation, with gliogenic, rather than neurogenic, potential, revealed under basal conditions. Three lines of evidence suggest that local FGF signalling governs α-tanycyte behaviour. First, we observe highly localised expression of endogenous Fgf s in β- and ventral α2-tanycytes. Second, blockade of FGF signalling ex vivo significantly reduces basal α-tanycyte proliferation; similarly, α-tanycyte-derived neurospheres are dependent upon FGF for self-renewal in vitro . Third, α2-tancytes respond to elevated levels of FGF in vivo through enhanced proliferation. FGFs and FGF receptors have been described in other adult NSC niches, and are widely accepted to be potent modulators of progenitor cell proliferation, but in neither the SVZ nor the SGZ do they display a highly localised distribution [44] , [45] . The presence of endogenous Fgf s and evidence of the requirement for active growth factor signalling suggest that FGF signalling has a role in the control of α-tanyctes under normal conditions, perhaps limiting differentiation that might occur through localised CNTF [1] , [46] . Our finding that α-tanycytes give rise to β-tanycytes that may themselves express Fgf-10 (this study and Haan et al. [23] ) suggests a mechanism for maintaining Fgf levels in the niche. The IIIc isoforms of FGFR1 and FGFR2, which have high affinity for FGF-2 and FGF-18 [47] , [48] , are detected in the central/posterior hypothalamus [12] , supporting the idea that FGF-18 at least may act as an endogenous regulator of cellular homeostasis in the hypothalamus. It remains to be seen if FGFs or other trophic factors mediate the proliferative response of α-tanycytes to dietary or other environmental challenges. Our findings into the identification of a novel hypothalamic stem cell and its regulation have potential implications for homeostatic functions. Our previous studies [1] and those of others [6] , [11] , [12] , [23] show that new cells, including neurons, can be generated in the adult mouse hypothalamus, and reveal a cellular dynamism in the postnatal/adult hypothalamus in response to altered signalling (this study and those of others [5] , [7] ). Our study provides an indication that FGF signalling governs self-renewal of a hypothalamic NSC, and suggests that adult α2-tanycytes, known to act as a bridge between the cerebrospinal fluid/portal blood supply and neurons in hypothalamic nuclei, might mediate long-term physiological effects via their capacity to act as a NSC. Animals Mice were 8–12-week-old C57/Bl6, except for the NPY-GFP mice (a kind gift from Dr Brad Lowell, MGI Accession ID: MGI:3709062). GLAST::CreER T2 and Rosa26R mice have been described elsewhere [27] , [28] , [29] . BrdU analyses were approved by the institutional animal care and use committee of Beth Israel Deaconess Medical Center; lineage-tracing studies were conducted according to Max Planck institutional and German Federal regulations (licence numbers H-05/01, 0-06/02, G-09/18 and G-09/19). Neurosphere cultures Mice were killed, and the hypothalamus (or relevant subdissections) dissected out, minced, incubated in TrypLE enzyme solution (Calbiochem) for 20 min at 37 °C, then mechanically dissociated using a sequence of 25-gauge and 30-gauge needles. The resulting single-cell suspensions were plated at 10 cells/microlitre in ultra-low binding 24-well plates (Corning), in DMEM:F12 (Invitrogen) supplemented with penicillin/streptomycin, L-glutamine, B27, modified N2, progesterone, selenite, putrescine, transferrin, insulin-like growth factor 1, and 20 ng ml −1 each of EGF and FGF-2 (Fisher). Cultures were incubated in humidified chambers with 5% CO 2 at 37 °C. Neurosphere growth was assessed 10 days after plating. Neurospheres were passaged by incubating for 20 min in TrypLE solution, before mechanically dissociating the spheres into a single-cell suspension, and plating as per the original conditions. Differentiation of neurospheres was performed in 8-well chamber slides (SLS). They were coated with 150 μg ml −1 poly-D-lysine (Sigma) and 100 μg ml −1 Fibronectin (Sigma) prior to use. The same basic medium as used for neurosphere growth was used, but containing 10 ng ml −1 of FGF-2 and no EGF. A single neurosphere was transferred to each chamber and incubated for 7 days before fixation and processing. Tamoxifen-induced Cre labelling Stock solutions of Tamoxifen (Sigma) were prepared at a concentration of 20 mg ml −1 in corn oil (Sigma). Mice were injected i.p. with Tamoxifen once per day for 10 consecutive days at a dose of 2 mg per day. β-Gal expression was detected either by X-gal staining (1 mg ml −1 , Sigma) of cryosections [49] or by immunostaining with rabbit anti-β-Gal antibodies (1:2,000; Cappel). FGF-2 and BrdU infusions Mice were stereotactically implanted with a steel guide cannula into the right lateral cerebroventricle. The cannula was connected to an osmotic minipump and the mice were infused for 7 days. The vehicle solution was aCSF containing 1 μg μl −1 mouse serum albumin (Sigma, St Louis, MO, USA) and 1 μg μl −1 5-bromodeoxyuridine (BrdU, Sigma) [1] . FGF-2 (R&D systems) was used at a concentration of 64.8 ng μl −1 . Mice were harvested either acutely or 6 weeks following the start of infusion. Each group consisted of six animals. Mice were perfused with 10% formalin and cut into 14 μM coronal sections using a cryostat. Tissues were treated with 2N HCl for 1 h to expose the BrdU antigen, and were then processed for antibody labelling. Immunohistochemistry Mice were perfused with 4% paraformaldehyde (PFA); neurospheres were fixed in either 4% PFA or MEMFA. Tissues/cells were immersed in 30% sucrose and cut into 12–20 μM coronal sections using a cryostat, then incubated in primary antibody diluted in PBS+1–3% serum+0.1% Triton X-100 overnight. A solution of secondary antibody was then applied for 30–180 min at RT, with 4′,6-diamidino-2-phenylindole (DAPI) added to visualise the cell nuclei. In the cases of Vimentin and Nestin, heat-mediated antigen retrieval in citrate buffer was performed. The following primary antibodies were used: GFAP (1:200, Chemicon or 1:50, BD Pharmingen), Nestin (1:200 Chemicon), MAP2 (1:1,000, Sigma), RIP (1:10, DS Hybridoma Bank), TuJ1 (1:1,000, Calbiochem), HuC/D (1:70, Molecular Probes), pErk1/2 (1:50, Cell Signalling Technologies), Sox2 (1:200, Chemicon), BrdU (1:200, Accurate), AVP (1:500, gift from H. Kawana) and Vimentin (1:200 Sigma). Secondary antibodies were conjugated to either FITC, Cy3 or Dylight649 (1:200, Jackson Immunoresearch) or Alexa488 or Alexa594 (1:500, Molecular Probes). Organotypic slice culture Mice were killed and the hypothalamus was dissected in ice-cold L-15 to be subsequently mounted in 3% agarose/HBSS. A vibratome was used to obtain 200-μm hypothalamic slices in ice-cold L-15. Tuberal slices were embedded in collagen/DMEM and incubated at 5% CO 2 and 37 °C in neurosphere medium, as described above, minus insulin/IGF-1, for a 24-h recovery period. Experimental treatments were applied for 24 h following the recovery period, FGF-2 (Sigma, 20 ng ml −1 ), SU5402 (Millipore, 6 ng ml −1 ) and vehicle (DMSO). In situ hybridisation Mice were perfused with 4% PFA, brains removed and cut into 30-μM coronal sections using a cryostat. Sections were permeabilized with proteinase K, acetylated, and then hybridised with DIG-labelled RNA probes overnight at 68 °C. Signals were revealed using alkaline phosphatase-conjugated antibodies to DIG (1:2,000, Roche) and nitroblue tetrazolium chloride/5-bromo-4-chloro-3-indolyl-phosphate. RT–PCR RNA was extracted from high-passage neurospheres using a commercial kit (Stratagene). Two micrograms of RNA were then used for reverse transcription reactions using the manufacturer’s protocol for SuperScript III Reverse Transcriptase (Invitrogen). Samples were run for 32 cycles using an annealing temperature of 55 °C, and then run on a 1% agarose gel to confirm whether the product was of the correct size. RT–PCR was performed with primers specific for FGF-10 (forward primer: GCCACCAACTGCTCTTCTTC, reverse primer: CTCTCCTGGGAGCTCCTTTT) and FGF-18 (forward primer: CCTGCACTTGCCTGTGTTTA, reverse primer: AGCCCACATACCAACCAGAG). Imaging Immunohistological Imaging was carried out on either using an Axio Imager.A1 microscope (Zeiss) or subjected to three-dimensional reconstruction using a LSM 510 META upright confocal microscope (Zeiss). Images were processed with Adobe Photoshop 7.0 software (Adobe Systems, San Jose, CA, USA). How to cite this article: Robins, S. C. et al. α-Tanycytes of the adult hypothalamic third ventricle include distinct populations of FGF-responsive neural progenitors. Nat. Commun. 4:2049 doi: 10.1038/ncomms3049 (2013).